Sas-4 provides a scaffold for cytoplasmic complexes and tethers them in a centrosome Centrosomes are conserved organelles that are essential for accurate cell division and cilium formation. A centrosome consists of a pair of centrioles surrounded by a protein network of pericentriolar material (PCM) that is essential for the centrosome's function. In this study, we show that Sas-4 provides a scaffold for cytoplasmic complexes (named S-CAP), which include CNN, Asl and D-PLP, proteins that are all found in the centrosomes at the vicinity of the centriole. When Sas-4 is absent, nascent procentrioles are unstable and lack PCM, and functional centrosomes are not generated. When Sas-4 is mutated, so that it cannot form S-CAP complexes, centrosomes are present but with dramatically reduced levels of PCM. Finally, purified S-CAP complexes or recombinant Sas-4 can bind centrosomes stripped of PCM, whereas recombinant CNN or Asl cannot. In summary, PCM assembly begins in the cytosol where Sas-4 provides a scaffold for pre-assembled cytoplasmic complexes before tethering of the complexes in a centrosome. The centrosome consists of a pair of centrioles surrounded by an amorphous protein network of pericentriolar material (PCM). The PCM must assemble around a centriole, as the PCM is necessary for the resulting centrosome to function by serving as the principal site for microtubule nucleation and anchoring [1] , [2] , [3] , [4] . Additionally, formation of a daughter centriole occurs in the PCM, with the PCM appearing to have essential roles in this process [2] , [5] . The importance of the PCM to the fate of a cell and the organism itself is well documented [6] . Although several complexes of PCM components have been identified [7] , [8] , the mechanism by which PCM is assembled to generate a normally functioning centrosome is unclear. Asterless (Asl) is a centriole duplication factor that has long been thought to have a key role in PCM assembly [9] , [10] , [11] , [12] , this is concordant with the observation that Asl co-localizes with Sas-4, CNN and D-PLP at the vicinity of the centriole [12] , [13] , [14] , [15] , [16] , [17] , [18] , [19] . However, in vitro , when Asl is partially depleted, centrosomes are observed that contain Sas-4 (ref. 20 ). Similarly, in vivo , Asl appears to have only a small effect on PCM assembly; instead it is essential for centriole duplication [14] . As it is likely that Asl has only a secondary role in PCM assembly in vivo , the specific protein that is responsible for recruiting PCM proteins to a centriole remains unknown. Sas-4 and its human orthologue CPAP are known to form complexes with tubulin and γ-tubulin and are essential for centrosome biogenesis [19] , [21] , [22] , [23] , [24] . Reduced amounts of Sas-4 result in centrosomes that contain less PCM, and an absence of Sas-4 prevents the maturation of a centrosome from a nascent procentriole (an early centriolar intermediate without microtubules) [23] , [25] , [26] . In contrast, overexpression of Sas-4 or CPAP results in acentriolar centrosomes [27] or in elongated centrioles that have assembled PCM [28] , [29] , [30] , [31] . The formation of the elongated centrioles is dependent on tubulin binding to a conserved segment in the Sas-4 domain known as PN2-3 (refs 21 , 22 , 28 ). Ultrastructurally, Sas-4/CPAP is observed at the centriole and in the PCM [19] , [23] , [25] , [32] . Accordingly, it is likely that Sas-4 serves pivotal roles in both centriole formation and PCM assembly, yet how Sas-4 accomplishes these roles are currently unclear. In this study, we investigated the role of Sas-4 in scaffolding cytoplasmic complexes and show that it is required for the incorporation of PCM into centrioles. The localization of Sas-4 suggests a role in pericentriolar material assembly To aid our studies, we generated an anti-Sas-4 monoclonal antibody ( Supplementary Fig. S1a,b ). Using this antibody, we studied Sas-4's localization in centrosomes of various Drosophila cell types. In embryonic cells, the anti-Sas-4 antibody labels centrosomes ( Fig. 1a ). In early and intermediate spermatocytes, Sas-4 is present along the entire length of a centrosome. In mature spermatocytes and early spermatids, Sas-4 is restricted to the proximal end of a centrosome ( Fig. 1b ). This pattern supports the premise that Sas-4 functions in PCM assembly, which is known to begin at the proximal end of a centrosome [33] . 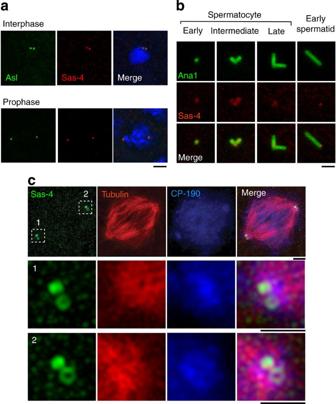Figure 1: Centrosomal localization ofDrosophilaSas-4. (a) The anti-Sas-4 antibody labels embryonic centrosomes. Centrosomes are marked by Asl-GFP. Blue, DAPI. Scale bar, 2 μm. (b) Sas-4's location in sperm centrosomes varies over development. Ana1-GFP, a centriolar marker, labels centrosomes. Scale bar, 1 μm. (c) Sas-4 labels a 'toroid-shaped' structure around the centriole core. 3D-structured illumination microscopy of Sas-4-labelled (green) mitotic centrosomes inDrosophilaS2 cells (Supplementary Fig. S1). Tubulin (red) and CP-190 (blue) mark the PCM. Scale bars are 1 μm. Figure 1: Centrosomal localization of Drosophila Sas-4. ( a ) The anti-Sas-4 antibody labels embryonic centrosomes. Centrosomes are marked by Asl-GFP. Blue, DAPI. Scale bar, 2 μm. ( b ) Sas-4's location in sperm centrosomes varies over development. Ana1-GFP, a centriolar marker, labels centrosomes. Scale bar, 1 μm. ( c ) Sas-4 labels a 'toroid-shaped' structure around the centriole core. 3D-structured illumination microscopy of Sas-4-labelled (green) mitotic centrosomes in Drosophila S2 cells ( Supplementary Fig. S1 ). Tubulin (red) and CP-190 (blue) mark the PCM. Scale bars are 1 μm. Full size image To determine the fine localization of Sas-4 in a centrosome, we used three-dimensional (3D) structured illumination microscopy [34] and immuno-electron microscopy. When mitotic centrosomes are visualized using 3D-structured illumination microscopy, Sas-4 labelling has a toroid shape, surrounding what is likely to be a centriole. Therefore, Sas-4 appears to be at the vicinity of a centriole ( Fig. 1c ). Similarly, pre-embedding immuno-electron microscopy of isolated centrosomes shows that Sas-4 is located at the internal and external surfaces of the centriole wall and in the PCM ( Supplementary Fig. S2 ). Thus, Sas-4 is in a position that would allow it to tether PCM proteins to a centriole. Sas-4 is present in cytoplasmic complexes To determine whether Sas-4 interacts with proteins that eventually are found at the vicinity of the centriole, first we conducted a preliminary characterization of Sas-4's biochemical relationship with PCM and centrosomes using linear sucrose-gradient velocity sedimentation of embryonic extracts. Under low-salt conditions, centrosomes, which include the centriolar proteins Sas-6 and Ana1 and the PCM proteins Asl, CNN and γ-tubulin are detected in high-density sedimentation fractions and cytoplasmic PCM proteins are detected in the low-density fractions [7] , [8] , [35] . Moreover, under high-salt conditions, PCM proteins are found only in the low-density (cytoplasmic) fractions, whereas the centriolar proteins remain in the high-density fractions [14] , [35] , [36] . In other words, high salt removes PCM proteins from a centrosome, leaving a 'stripped-centrosome'. When we fractionate embryonic extracts under low-salt conditions, Sas-4 and D-PLP co-fractionate in both the centrosomal and cytoplasmic fractions ( Supplementary Fig. S3a ). However, under high-salt conditions, Sas-4 and D-PLP are only in the cytoplasmic fractions ( Supplementary Fig. S3b ), indicating that these proteins were stripped from centrosomes. Thus, these proteins may associate both in centrosomes and in the cytoplasm. The observation that Sas-4 and D-PLP respond to salt conditions and fractionate similar to the response reported for CNN, Asl and γ-tubulin supports the idea that they are either part of the same complex or are components of different complexes with similar biochemical properties. To identify proteins that interact with Sas-4 in vivo , we purified Sas-4-containing complexes from embryonic extracts and analysed their composition. First, high-speed lysates (HSLs), which lack centrosomes, were prepared ( Supplementary S4a,b ). Next, the cytoplasmic Sas-4-containing complexes were immuno-precipitated from the HSLs using our anti-Sas-4 antibody ( Supplementary Fig. S4a ). Thereafter, mass-spectrometry was performed on the Sas-4 precipitates ( Supplementary Fig. S5a ). Finally, a list of putative Sas-4-interacting proteins was obtained by subtracting the results from Sas-6-interacting proteins (centriolar proteins) and from the empty beads control ( Supplementary Fig. S5b ). The list of putative Sas-4-interacting proteins includes CNN, D-PLP and CP-190 ( Supplementary Fig. S5b ). Western blots confirm that these proteins are present in the Sas-4-precipitated complexes and that Asl is also present in the complex ( Fig. 2a ; Supplementary Fig. S4c ). Similar results were obtained using affinity-purified complexes from Sas-4-TAP-expressing embryos ( Fig. 2b ). Therefore, Sas-4 is present in cytoplasmic complexes that include proteins that are present at the vicinity of the centriole. 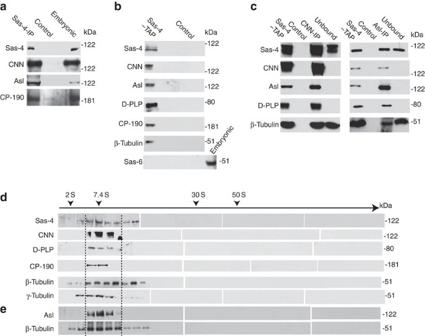Figure 2: Sas-4 is present in cytoplasmic complexes. (a) Immunoprecipitations using the anti-Sas-4 antibody of HSLs reveal associations between Sas-4 and other proteins. Embryonic extracts were used as the positive control; uncoated beads were used as the negative control (Control). (b) CNN, Asl, D-PLP, CP-190 and β-tubulin co-purify with Sas-4 in tandem affinity purification (TAP) of HSL from Sas-4–TAP-expressing embryos (Sas-4–TAP). The centriolar protein Sas-6 was only detected in embryonic extracts. (c) CNN (CNN-IP) or Asl (Asl-IP) co-immunoprecipitates Sas-4, D-PLP and tubulin from the TAP-purified Sas-4-containing complexes (Sas-4–TAP). A portion of the TAP-purified Sas-4-containing complexes was not precipitated by the antibody-coated beads (Unbound), which contains Sas-4 and tubulin. None of the above proteins is detected from uncoated beads (Control). (d,e) TAP-purified Sas-4-containing complexes fractionate around 7 S in a 15–60% sucrose gradient. (d) Whereas Sas-4, β-tubulin and γ-tubulin are widely distributed, CNN, D-PLP and CP-190, were restricted to only a narrow range of fractions (∼7 S). (e) Asl was also detected as a narrow distribution in experiments that included nocodozole (100 ng ml−1) which inhibits microtubule polymerization. Figure 2: Sas-4 is present in cytoplasmic complexes. ( a ) Immunoprecipitations using the anti-Sas-4 antibody of HSLs reveal associations between Sas-4 and other proteins. Embryonic extracts were used as the positive control; uncoated beads were used as the negative control (Control). ( b ) CNN, Asl, D-PLP, CP-190 and β-tubulin co-purify with Sas-4 in tandem affinity purification (TAP) of HSL from Sas-4–TAP-expressing embryos (Sas-4–TAP). The centriolar protein Sas-6 was only detected in embryonic extracts. ( c ) CNN (CNN-IP) or Asl (Asl-IP) co-immunoprecipitates Sas-4, D-PLP and tubulin from the TAP-purified Sas-4-containing complexes (Sas-4–TAP). A portion of the TAP-purified Sas-4-containing complexes was not precipitated by the antibody-coated beads (Unbound), which contains Sas-4 and tubulin. None of the above proteins is detected from uncoated beads (Control). ( d , e ) TAP-purified Sas-4-containing complexes fractionate around 7 S in a 15–60% sucrose gradient. ( d ) Whereas Sas-4, β-tubulin and γ-tubulin are widely distributed, CNN, D-PLP and CP-190, were restricted to only a narrow range of fractions ( ∼ 7 S). ( e ) Asl was also detected as a narrow distribution in experiments that included nocodozole (100 ng ml −1 ) which inhibits microtubule polymerization. Full size image To test whether Sas-4 forms one or more complexes, we immunoprecipitated Sas-4 complexes using anti-CNN or anti-Asl antibodies ( Fig. 2c ). Both CNN- and Asl-precipitated complexes contain Sas-4, CNN, Asl, D-PLP and β-tubulin; in contrast, the fraction not bound by the anti-CNN or anti-Asl antibodies contains β-tubulin and Sas-4 but lacks CNN, Asl and D-PLP ( Fig. 2c ). Accordingly, Sas-4 exists in at least two distinct groups of complexes: those with tubulin but not CNN, D-PLP or CP-190 and those with tubulin and CNN, Asl, D-PLP and CP-190. We further characterized the purified cytoplasmic Sas-4 complexes by velocity sedimentation ( Fig. 2d,e ). The purified complexes fractionate with a sedimentation coefficient starting around 7 S, which is the same as the coefficient for complexes obtained from embryonic extracts ( Supplementary Fig. S3a ). Corroborating our western blot data, we find that CNN, Asl, D-PLP and CP-190 co-fractionate with Sas-4 in a narrow range of fractions ( Fig. 2d,e : between dotted lines), further demonstrating that these proteins are in the same complexes. In contrast, β-tubulin and γ-tubulin co-fractionate with Sas-4 in a wide range of fractions ( Fig. 2d ). Under conditions that inhibit microtubule polymerization, a similarly wide range of β-tubulin-containing fractions is obtained, indicating that Sas-4 and β-tubulin, and possibly γ-tubulin, exist in multiple, different-sized complex types ( Fig. 2e ). These data reveal that in vivo Sas-4 simultaneously interacts with at least CNN, Asl, and D-PLP, in cytoplasmic 'S-CAP complexes'; further analysis of the S-CAP complexes may elucidate how those proteins are transported from the cytoplasm and become co-localized at the centriole. Sas-4 is essential for PCM recruitment We then asked whether the proteins that are normally present in an S-CAP complex could be recruited to a nascent procentriole, the structure that forms in the absence of Sas-4 (refs 26 , 37 ). For this, we analysed recruitment of S-CAP complex components in sas-4 null ( sas-4 s2214 ) pupae at a developmental stage when maternally contributed Sas-4 has been depleted [24] . Stem cells in the testes of centrosomal mutants appear to have normal centrosomes, as these centrosomes are formed using maternally contributed proteins [14] , [38] . Indeed, electron microscopy analyses of sas-4 s2214 testes reveal that only cells in the stem cell region appear to have normal centrioles [39] . To avoid analysing these maternally contributed centrosomes in sas-4 s2214 flies, we used a FasIII antibody to mark the stem cell region; in these experiments, we specifically excluded these maternally contributed centrosomes found in the FasIII-positive region [38] . To mark the nascent procentrioles in sas-4 s2214 flies, we used pupae that synthesize Sas-6-GFP or Ana1-GFP [26] , [37] . Note that sas-6-GFP or ana1-GFP expression was regulated by native sas-6 or ana1 promoters and was expressed at near physiological levels ( Supplementary Fig. S6a ). Consequently, it is unlikely that these fusion proteins would produce the artificial centriolar structures that are observed when centriolar proteins are strongly overexpressed [27] , [36] , [40] , [41] . In control pupae, which produce wild-type Sas-4, Ana1 labelling is found in centrosomes of sperm cells at all developmental stages; this includes the centrosomes of spermatogonium and elongated centrosomes of matured spermatocytes ( Fig. 3a ). In contrast, sas-4 s2214 pupae display Ana1 labelling only in spermatogonia (away from the FasIII-labelled stem cell region) and not in later-stage spermatocytes ( Fig. 3a ). Most significantly, we found that although the sas-4 s2214 pupae contain the centriolar proteins Sas-6 and Ana1, they lack S-CAP proteins that co-immunoprecipitate with Sas-4 ( Fig. 3b–e ; Supplementary Fig. S6 ). Together, in the absence of Sas-4, nascent procentrioles fail to recruit the S-CAP complex components; however, it is possible that the failure of S-CAP complex recruitment is due to the absence of normal centrioles in the sas-4 -null mutants. 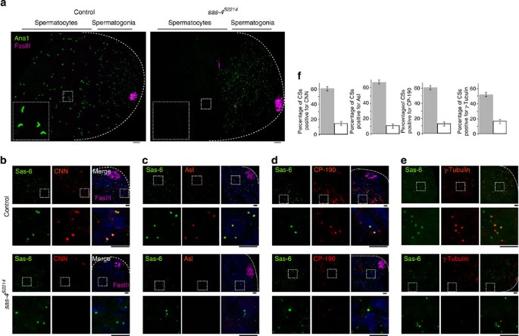Figure 3: Nascent procentrioles inSas-4mutants are transiently present and lack PCM. (a) In control testes, developing and elongated centrioles are labelled by Ana1-GFP throughout the testis. The elongated centrioles within the dashed box are enlarged in the inset. InSas-4s2214-null mutants, Ana1-GFP only labels nascent centrioles present in spermatogonia; Ana1-GFP is absent from differentiating spermatocyte cells. Dotted lines mark a testis' boundaries. In this analysis, we excluded the maternally contributed centrioles that are restricted to the stem cells, identified by Fas III (magenta) labelling23,36,38. Scale bar, 10 and 2 μm for higher and lower magnification, respectively. (b–f) In early differentiating sperm cells, centriolar structures in control testes andSas-4s2214-null mutant testes are labelled by Sas-6-GFP. CNN (b), Asl (c), CP-190 (d) and γ-tubulin (e) are present in control centrioles but not inSas-4s2214nascent procentrioles. Dashed boxes mark the enlarged areas shown in the lower panels. Scale bar, 2 μm. (f) Charts showing the fraction of centriolar structures (CSs) that are positive for each PCM protein in the control (grey filling) and inSas-4s2214(white filling); for each chart, Sas-6-GFP-labelled CSs were counted within a 20 μm2area that is 10 μm from the stem cell region or∼25 μm from the tip of a testis (dotted lines). The mean±s.e.m. of six independent testes are shown. Figure 3: Nascent procentrioles in Sas-4 mutants are transiently present and lack PCM. ( a ) In control testes, developing and elongated centrioles are labelled by Ana1-GFP throughout the testis. The elongated centrioles within the dashed box are enlarged in the inset. In Sas-4 s2214 -null mutants, Ana1-GFP only labels nascent centrioles present in spermatogonia; Ana1-GFP is absent from differentiating spermatocyte cells. Dotted lines mark a testis' boundaries. In this analysis, we excluded the maternally contributed centrioles that are restricted to the stem cells, identified by Fas III (magenta) labelling [23] , [36] , [38] . Scale bar, 10 and 2 μm for higher and lower magnification, respectively. ( b – f ) In early differentiating sperm cells, centriolar structures in control testes and Sas-4 s2214 -null mutant testes are labelled by Sas-6-GFP. CNN ( b ), Asl ( c ), CP-190 ( d ) and γ-tubulin ( e ) are present in control centrioles but not in Sas-4 s2214 nascent procentrioles. Dashed boxes mark the enlarged areas shown in the lower panels. Scale bar, 2 μm. ( f ) Charts showing the fraction of centriolar structures (CSs) that are positive for each PCM protein in the control (grey filling) and in Sas-4 s2214 (white filling); for each chart, Sas-6-GFP-labelled CSs were counted within a 20 μm 2 area that is 10 μm from the stem cell region or ∼ 25 μm from the tip of a testis (dotted lines). The mean±s.e.m. of six independent testes are shown. Full size image To determine the specific role of Sas-4 in S-CAP complex formation, we overexpressed Sas-4 in S2 cells. We find that Sas-4 overexpression induces numerous cytoplasmic Sas-4-positive foci per cell, with most cells having greater than four foci per cell ( Fig. 4a–d ). The two foci found in control cells (along with the extra foci seen in Sas-4-overexpressing cells) contain both S-CAP complex components and the centriole-specific marker Ana1, indicating that these foci are native centrosomes ( Fig. 4a–d ). In contrast, the Sas-4-induced foci contain the S-CAP complex components yet lack any centriolar proteins ( Fig. 4d,e ). We then analysed the Sas-4-induced foci using velocity sedimentation. Extracts of Sas-4-overexpressing cells contain an intermediate-density fraction that is absent from untransfected cells ( Fig. 4f ); this intermediate fraction is significantly denser than native cytoplasmic complexes. Additionally, the sedimentation pattern of the centriolar protein Sas-6 (refs 36 , 43 ) remains unchanged in both untransfected and Sas-4-overexpressing cells. These data, along with the finding that the Sas-4-induced foci lack the centriolar protein Ana1 (ref. 37 ), indicate that the these foci are not additional centrosomes but rather aggregates of S-CAP complexes. 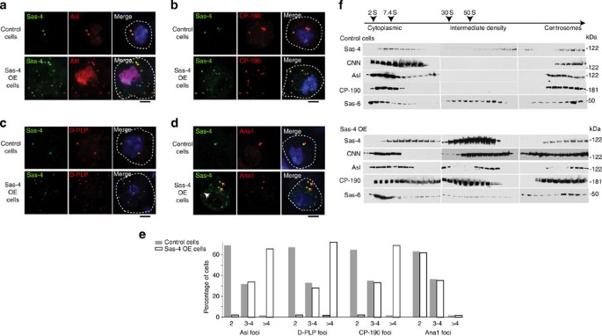Figure 4: Overexpression of Sas-4 inDrosophilacells induces foci containing S-CAP components. (a–d) Sas-4-GFP overexpression (OE) in S2 cells induces foci that contain Asl (a), D-PLP (b) and CP-190 (c) but not the centriolar protein Ana1 (d). In (d), yellow arrows point out the Sas-4- and Ana1-positive centrioles; the white arrow points out a Sas-4-positive but Ana1-negative focus. This is an example of a focus that was induced by Sas-4 OE. In (a), the nuclear Asl staining is nonspecific. Scale bar, 1 μm. (e) Quantification of control (grey filling) and Sas-4-GFP-induced (white filling) foci shown in panels (a–d) (n=50 except for Ana1, wheren=20). Note that∼30% of the S2 cells normally possess three to four centrioles per cell. (f) Velocity sedimentation of Sas-4-induced foci. Extracts of un-transfected control cells and Sas-4-transfected cells were separated on a 15–60% sucrose gradient. The intermediate density fractions induced by Sas-4 OE are not detected in control cells. The Sas-4-induced foci co-fractionate with CNN, Asl and CP-190. The fractionation pattern of the centriole core-specific protein Sas-6 remained unchanged in both control cells and Sas-4-transfected cells. Figure 4: Overexpression of Sas-4 in Drosophila cells induces foci containing S-CAP components. ( a – d ) Sas-4-GFP overexpression (OE) in S2 cells induces foci that contain Asl ( a ), D-PLP ( b ) and CP-190 ( c ) but not the centriolar protein Ana1 ( d ). In ( d ), yellow arrows point out the Sas-4- and Ana1-positive centrioles; the white arrow points out a Sas-4-positive but Ana1-negative focus. This is an example of a focus that was induced by Sas-4 OE. In ( a ), the nuclear Asl staining is nonspecific. Scale bar, 1 μm. ( e ) Quantification of control (grey filling) and Sas-4-GFP-induced (white filling) foci shown in panels ( a – d ) ( n =50 except for Ana1, where n =20). Note that ∼ 30% of the S2 cells normally possess three to four centrioles per cell. ( f ) Velocity sedimentation of Sas-4-induced foci. Extracts of un-transfected control cells and Sas-4-transfected cells were separated on a 15–60% sucrose gradient. The intermediate density fractions induced by Sas-4 OE are not detected in control cells. The Sas-4-induced foci co-fractionate with CNN, Asl and CP-190. The fractionation pattern of the centriole core-specific protein Sas-6 remained unchanged in both control cells and Sas-4-transfected cells. Full size image The N-terminal domain of Sas-4 is essential for complex formation We then began our analysis to understand the mechanism of S-CAP complex formation. We first searched for the domain in Sas-4 that is essential for its interaction with S-CAP complex components. To this end, we generated GFP-tagged, truncated versions of Sas-4 and screened for a domain that is required for assembling S-CAP complexes, using D-PLP's localization as a marker ( Supplementary Fig. S7a ). As expected, full-length Sas-4 is localized to centrosomes and induces foci that include D-PLP. In contrast, variants that lack either the first 150 or 350 residues of Sas-4 (Sas-4Δ150 and Sas-4Δ350, respectively) can induce foci, which fail to include D-PLP. These suggest that residues 1–150 are required for Sas-4's interaction with D-PLP and possibly for Sas-4's assembly of S-CAP complexes. Nonetheless, Sas-4Δ150 and Sas-4Δ350 are localized to centrosomes, indicating that the region of Sas-4 that primarily interacts with centrosomes is located in its C-terminus. In agreement with these findings, Sas-4 variants that include the first 150 residues of Sas-4, but lack residues beyond position 350 (Sas-4-N and Sas-4-N350), are diffused throughout the cytoplasm. Second, we investigated the ability of Sas-4's N-terminal domain to bind other components of the S-CAP complex. We performed co-immunoprecipitation of HSLs from S2 cells using Sas-4 or Sas-4Δ150 as bait ( Fig. 5a ). As expected, Sas-4 precipitates CP-190, CNN and β-tubulin ( Fig. 5b ). In contrast, Sas-4Δ150 precipitates CP-190 but not CNN or β-tubulin, suggesting that Sas-4's N-terminal is necessary for, at least, CNN and tubulin binding ( Fig. 5b ). Next, we tested the sufficiency of the N-terminal domain of Sas-4 in binding these S-CAP complex components. Sas-4-N is able to immunoprecipitate CNN and β-tubulin from S2 cells ( Fig. 5b ). Likewise, recombinant Sas-4 N-terminal domain (Sas-4-N190) pulls down CNN, Asl, D-PLP and β-tubulin from embryonic HSL ( Fig. 5c ). Finally, Sas-4-N190 and CNN directly interact via CNN's N-terminal half ( Fig. 5d ; Supplementary Fig. S8a ). In summary, the N-terminal domain of Sas-4 is necessary and sufficient for Sas-4's binding to the S-CAP complex components. 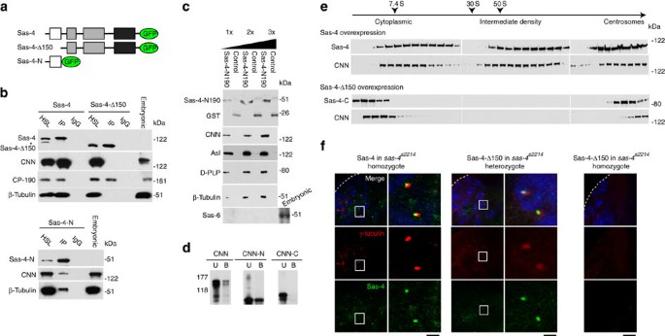Figure 5: The N-terminal domain of Sas-4 is necessary and sufficient for the assembly of S-CAP complexes. (a) Schematics of the Sas-4-containing, GFP-tagged constructs: Sas-4, Sas-4Δ150, and Sas-4-N. (b) Co-immunoprecipitation experiments using S2 cells that express Sas-4, Sas-4Δ150, or Sas-4-N. HSL, high-speed cell lysate; IP, immunoprecipitation; IgG, beads coated with a nonspecific mouse IgG; and Embryonic: embryonic extract. The asterisk marks a band that may be an isoform of Sas-4. (c) Sas-4-N190 (which includes only the first 190 amino acids of Sas-4) pulls down CNN, Asl, D-PLP and β-tubulin but not the centriolar-specific protein Sas-6 from embryonic HSL. The purified recombinant proteins used in this figure are shown inSupplementary Fig. S8. (d) Sas-4 binds directly to CNN via the N-terminal half of CNN. Anti-Sas-4 antibody-coated beads immobilized Sas-4-N190, which was used to bind CNN or its truncated variants. Sas-4-N190 binds purified full-length CNN (CNN) and CNN's N-terminal half. The C-terminal half of CNN (CNN-C) does not bind Sas-4-N190. B, bound; U, unbound. (e) The N-terminal domain of Sas-4 is essential in the formation of S-CAP complexes and Sas-4-induced foci. Comparison of fractionation patterns for S2 cell extracts transfected with either Sas-4 or Sas-4Δ150. (f) The N-terminal domain of Sas-4 is required for the formation of functional centrosomes. Analysed are testes of homozygousSas-4S2214-null mutants that have been transfected with Sas-4, heterozygousSas-4S2214mutants transfected with Sas-4Δ150, and homozygousSas-4S2214mutants transfected with Sas-4Δ150. The tip of a testis is marked with dotted lines. Scale bar, 10 and 2 μm for higher (left) and lower (right) magnification, respectively. Figure 5: The N-terminal domain of Sas-4 is necessary and sufficient for the assembly of S-CAP complexes. ( a ) Schematics of the Sas-4-containing, GFP-tagged constructs: Sas-4, Sas-4Δ150, and Sas-4-N. ( b ) Co-immunoprecipitation experiments using S2 cells that express Sas-4, Sas-4Δ150, or Sas-4-N. HSL, high-speed cell lysate; IP, immunoprecipitation; IgG, beads coated with a nonspecific mouse IgG; and Embryonic: embryonic extract. The asterisk marks a band that may be an isoform of Sas-4. ( c ) Sas-4-N190 (which includes only the first 190 amino acids of Sas-4) pulls down CNN, Asl, D-PLP and β-tubulin but not the centriolar-specific protein Sas-6 from embryonic HSL. The purified recombinant proteins used in this figure are shown in Supplementary Fig. S8 . ( d ) Sas-4 binds directly to CNN via the N-terminal half of CNN. Anti-Sas-4 antibody-coated beads immobilized Sas-4-N190, which was used to bind CNN or its truncated variants. Sas-4-N190 binds purified full-length CNN (CNN) and CNN's N-terminal half. The C-terminal half of CNN (CNN-C) does not bind Sas-4-N190. B, bound; U, unbound. ( e ) The N-terminal domain of Sas-4 is essential in the formation of S-CAP complexes and Sas-4-induced foci. Comparison of fractionation patterns for S2 cell extracts transfected with either Sas-4 or Sas-4Δ150. ( f ) The N-terminal domain of Sas-4 is required for the formation of functional centrosomes. Analysed are testes of homozygous Sas-4 S2214 -null mutants that have been transfected with Sas-4, heterozygous Sas-4 S2214 mutants transfected with Sas-4Δ150, and homozygous Sas-4 S2214 mutants transfected with Sas-4Δ150. The tip of a testis is marked with dotted lines. Scale bar, 10 and 2 μm for higher (left) and lower (right) magnification, respectively. Full size image Third, we tested the requirement of Sas-4's N-terminal domain in the formation of Sas-4 complexes. When extracts of S2 cells that overexpress Sas-4 were subjected to velocity sedimentation, Sas-4 and CNN are present in the low-, intermediate- and high-density fractions ( Fig. 5e ). However, when Sas-4Δ150 is overexpressed, the intermediate-density fractions are not detected ( Fig. 5e ). Thus, in the absence of the N-terminal domain, aggregates of S-CAP complex components are not induced. Consequently, the N-terminal domain of Sas-4 appears to be specifically necessary for the formation of S-CAP complexes. Given the significance of the N-terminal domain of Sas-4 in S-CAP complexes formation, we then tested the in vivo consequences of its absence on centrosome biogenesis. For this, we made flies that express Sas-4 or Sas-4Δ150 in the sas-4 s2214 -null mutant. Sas-4 but not Sas-4Δ150 rescues the sas-4 s2214 uncoordination phenotype ( Fig. 5f ); not surprisingly, Sas-4-rescued flies have functional centrosomes, which contain γ-tubulin ( Fig. 5f ). When Sas-4Δ150 is expressed in sas-4 s2214 heterozygotes, Sas-4Δ150 is associated with centrosomes ( Fig. 5f ). When Sas-4Δ150 is expressed in sas-4 s2214 homozygotes, γ-tubulin is not detected, indicating that there are no functional centrosomes ( Fig. 5f ); the absence of Sas-4Δ150 labelling suggests that Sas-4's N-terminal domain is essential for its binding to a nascent procentriole. Taken together, our data suggest that the N-terminal domain of Sas-4 is the scaffolding site for S-CAP complexes, and is required for centrosome biogenesis. Sas-4 PN2-3 is essential for S-CAP complex recruitment To determine the role of Sas-4 in PCM assembly independent of its function in centriole biogenesis, we built two more constructs that have deletions in the N-terminal domain of Sas-4: Sas-4Δ90, which lacks residues 1–90, and Sas-4ΔPN2-3, which lacks residues 103–121 (the 19 residues conserved in PN2-3 domain) [22] , [28] . Flies were produced that express either of the constructs under the regulation of a Sas-4 promoter. Sas-4Δ90 or Sas-4ΔPN2-3 only partially rescues the sas-4 s2214 phenotype of uncoordination, indicating that these deleted segments mediate aspects of Sas-4's N-terminal domain's function. However, although Sas-4Δ90 flies are able to walk almost normally ( Supplementary Movies 1 and 2 ), most Sas-4ΔPN2-3 flies cannot stand, arguing that the PN2-3 domain is especially critical ( Supplementary Movie 3 ). When we analyse these flies' testes, we find that, unlike sas-4 -null mutants, the Sas-4ΔPN2-3 or Sas-4Δ90 flies have normal numbers of centrosomes ( Fig. 6a ), indicating that neither the PN2-3 domain nor the first 90 amino acids of Sas-4 are essential for centrosome biogenesis. Importantly, we find that centrosomes in Sas-4Δ90 flies have normal levels of CNN and Asl recruitment ( Fig. 6a–c ), whereas Sas-4ΔPN2-3 flies have dramatically reduced amounts of these proteins in their centrosomes ( Fig. 6a,d ). These data suggest that Sas-4's PN2-3 domain is responsible for recruiting CNN and Asl to the centrosome. 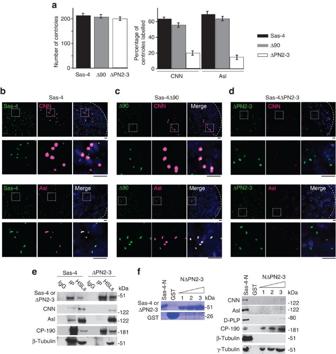Figure 6: S-CAP complex components bind to centrosomes via the PN2-3 domain of Sas-4. (a–d)In vivo, the PN2-3 domain is necessary for Sas-4's recruitment of S-CAP complex components to a centriole. (a) The number of centrioles observed at the tip of a testis (<60 μm from the hub) and the fractions of centrioles that are positive for CNN or Asl. The mean±s.e.m. of six independent testes are shown. (b,c) CNN and Asl are recruited to centrosomes of Sas-4s2214-null mutants that express Sas-4 or Sas-4Δ90. (d) In contrast, these proteins are not recruited to centrioles when Sas-4ΔPN2-3 is expressed. Dashed boxes mark the enlarged areas. Scale bar, 2 μm. (e)In vitro, the PN2-3 domain is necessary for Sas-4's binding to S-CAP complex components and their recruitment to a centriole. Co-immunoprecipitation experiments using extracts of S2 cells transfected with Sas-4 or Sas-4ΔPN2-3. In cells that overexpress Sas-4, CNN, Asl, CP-190, β-tubulin and γ-tubulin are immunoprecipitated (IP) from high-speed cell lysates (HSLs). In contrast, CP-190 and γ-tubulin but not CNN, Asl and β-tubulin are immunoprecipitated from HSLs of S2 cells that overexpress Sas-4ΔPN2-3. IgG: beads coated with a mouse IgG. (f) The PN2-3 domain of Sas-4 is required to pull down Asl, CNN or β-tubulin from embryonic HSLs. The purified recombinant proteins used are shown in Coomassie-stained gels. Sas-4-N–GST (which only includes the first 190 amino acids of Sas-4) pulls down Asl, CNN, β-tubulin, CP-190 and γ-tubulin from embryonic lysates. However, a Sas-4-N–GST variant, which lacks its PN2-3 domain ('NΔPN2-3'), can only pull down CP-190 and γ-tubulin. Figure 6: S-CAP complex components bind to centrosomes via the PN2-3 domain of Sas-4. ( a – d ) In vivo , the PN2-3 domain is necessary for Sas-4's recruitment of S-CAP complex components to a centriole. ( a ) The number of centrioles observed at the tip of a testis (<60 μm from the hub) and the fractions of centrioles that are positive for CNN or Asl. The mean±s.e.m. of six independent testes are shown. ( b , c ) CNN and Asl are recruited to centrosomes of Sas-4 s2214 -null mutants that express Sas-4 or Sas-4Δ90. ( d ) In contrast, these proteins are not recruited to centrioles when Sas-4ΔPN2-3 is expressed. Dashed boxes mark the enlarged areas. Scale bar, 2 μm. ( e ) In vitro , the PN2-3 domain is necessary for Sas-4's binding to S-CAP complex components and their recruitment to a centriole. Co-immunoprecipitation experiments using extracts of S2 cells transfected with Sas-4 or Sas-4ΔPN2-3. In cells that overexpress Sas-4, CNN, Asl, CP-190, β-tubulin and γ-tubulin are immunoprecipitated (IP) from high-speed cell lysates (HSLs). In contrast, CP-190 and γ-tubulin but not CNN, Asl and β-tubulin are immunoprecipitated from HSLs of S2 cells that overexpress Sas-4ΔPN2-3. IgG: beads coated with a mouse IgG. ( f ) The PN2-3 domain of Sas-4 is required to pull down Asl, CNN or β-tubulin from embryonic HSLs. The purified recombinant proteins used are shown in Coomassie-stained gels. Sas-4-N–GST (which only includes the first 190 amino acids of Sas-4) pulls down Asl, CNN, β-tubulin, CP-190 and γ-tubulin from embryonic lysates. However, a Sas-4-N–GST variant, which lacks its PN2-3 domain ('NΔPN2-3'), can only pull down CP-190 and γ-tubulin. Full size image To investigate the role of the PN2-3 domain in CNN and Asl recruitment to centrosomes, we overexpressed Sas-4ΔPN2-3 in S2 cells and observed whether foci were induced. We find that Sas-4ΔPN2-3 induces foci that do not contain Asl or D-PLP ( Supplementary Fig. S7b ). Although CNN, Asl and β-tubulin are produced at normal levels in the Sas-4ΔPN2-3-overexpressing cells ( Fig. 6e ), when we immunoprecipitate Sas-4ΔPN2-3 from the HSLs, we find greatly reduced binding of CNN, Asl and β-tubulin ( Fig. 6e ). These results provide evidence that the PN2-3 domain of Sas-4 is involved in recruiting and binding CNN, Asl and β-tubulin into Sas-4 complexes. In contrast, we did not observe a reduction in the recruitment or binding of CP-190 when the PN2-3 domain was absent. We then tested whether recombinant Sas-4ΔPN2-3 could interact with S-CAP complex components from HSLs of embryo extracts. For this, we used a version of Sas-4 that is truncated at residue 190 and lacks PN2-3 (that is, Sas-4-N190ΔPN2-3). Consistent with our S2 cell overexpression and in vivo data, purified recombinant Sas-4-N190ΔPN2-3 pulls down CP-190 and γ-tubulin but not CNN, Asl, D-PLP or β-tubulin ( Fig. 6f ). The finding that a Sas-4 that lacks its PN2-3 cannot recruit and bind β-tubulin is expected as PN2-3 domains have been shown to bind tubulin [22] , [28] ; that Sas-4-N190ΔPN2-3 cannot recruit and bind CNN or Asl, indicates that PN2-3 also mediates the binding of these proteins to Sas-4 and to a centrosome. Together, these results argue that the PN2-3 domain of Sas-4 is required for binding CNN, Asl and tubulin in the cytoplasm, which allows these proteins to be recruited to a centriole as part of S-CAP complex. Also, as centrosomes are observed in the absence of the PN2-3 domain, it appears that Asl present within an S-CAP complex has a centrosomal function other than in centriole formation. The function of the Asl that is bound to Sas-4 may be related to PCM morphology or its quantity [9] , [12] , [14] . S-CAP complexes bind to centrosomes stripped of PCM To understand how S-CAP complexes are bound in the centrosome, we designed experiments that reconstitute steps in this process in a cell-free system. It is known that high salt removes PCM components from a centrosome, leaving a 'stripped centrosome' that consists of a centriole and a salt-stable centrosome matrix [3] , [44] . With this in mind, we prepared stripped centrosomes from embryonic extracts using velocity sedimentation under a salt concentration of 500 mM KCl [14] , [36] , [45] . These stripped centrosomes contain a full complement of centriolar proteins but lack detectable levels of S-CAP complex components ( Fig. 7a ). We concurrently purified cytoplasmic S-CAP complexes from embryonic HSLs ( Fig. 7a ; Supplementary Fig. S9a ). We then tested whether these S-CAP complexes could bind to centrosomes or to stripped centrosomes in the cell-free system. S-CAP complexes were mixed with either type of centrosome and subjected to sucrose gradient velocity sedimentation ( Supplementary Fig. S9a ). This technique separates the mixtures into low-density fractions (which contain unbound S-CAP complexes) and high-density fractions (which contain stripped-centrosomes, with or without bound S-CAP complexes); these fractions were then analysed by western blotting. 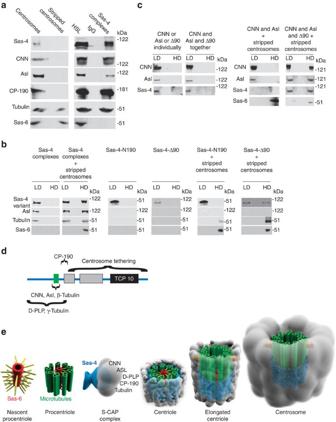Figure 7: S-CAP complexes bind to stripped centrosomes via Sas-4. (a) Centrosomes purified from wild-type embryonic extracts contain Sas-4, CNN, Asl, CP-190, tubulin and Sas-6, while stripped centrosomes contain only Sas-6 and tubulin. Purified Sas-4 complexes contain the Sas-4, CNN, Asl, CP-190 and tubulin. (b) Binding assays of purified Sas-4 complexes, Sas-4-N190 or Sas-4-Δ90 to stripped centrosomes and analyses by discontinuous sucrose gradient. Low-density (LD) fractions contain unbound proteins and high-density (HD) fractions contain stripped centrosomes and the proteins bound to them. In the absence of stripped centrosomes, Sas-4 complexes, Sas-4-N190 or Sas-4-Δ90 remain only in low-density fractions. When mixed with stripped centrosomes, Sas-4 complexes and Sas-4-Δ90 but not Sas-4-N190 are found in the HD fractions. Excess complexes and proteins remain in the unbound fractions. (c) Binding assays of Sas-4-Δ90, CNN or a combination of Sas-4-Δ90 and CNN to stripped centrosomes. LD fractions contain unbound proteins, whereas HD fractions contain stripped centrosomes and proteins bound to them. CNN or Asl alone cannot bind stripped centrosomes. In the presence of Sas-4-Δ90 and stripped centrosomes, CNN and Asl are bound to stripped centrosomes. (d) Schematic of the Sas-4 protein domains. Tethering: as Sas-4Δ90 binds to stripped centrosomes while Sas-4-N190 does not, the centrosome-binding domain of Sas-4 appears to be between residues 191 and 901. CNN, Asl, β-tubulin binding depends on the presence of the PN2-3 domain. D-PLP and γ-tubulin binding: as Sas-4-N190 binds to D-PLP and γ-tubulin, these proteins' binding domain in Sas-4 appears to be between residues 1 and 190. Green box: conserved segment in PN2-3 domain. CP-190 binding: as Sas-4-N190 and Sas-4Δ150 bind to CP-190, the CP-190 domain of Sas-4 appears to be between residues 151 and 190. (e) A model for the role of Sas-4 in PCM formation. Centrosome biogenesis begins with the formation of a nascent procentriole and the assembly of centriole microtubules. S-CAP complexes form in the cytoplasm and are then tethered to a procentriole via Sas-4. The centriole elongates and matures to a functional centrosome. Sas-4 (blue); microtubules (green); PCM (grey); appendages (orange). Figure 7: S-CAP complexes bind to stripped centrosomes via Sas-4. ( a ) Centrosomes purified from wild-type embryonic extracts contain Sas-4, CNN, Asl, CP-190, tubulin and Sas-6, while stripped centrosomes contain only Sas-6 and tubulin. Purified Sas-4 complexes contain the Sas-4, CNN, Asl, CP-190 and tubulin. ( b ) Binding assays of purified Sas-4 complexes, Sas-4-N190 or Sas-4-Δ90 to stripped centrosomes and analyses by discontinuous sucrose gradient. Low-density (LD) fractions contain unbound proteins and high-density (HD) fractions contain stripped centrosomes and the proteins bound to them. In the absence of stripped centrosomes, Sas-4 complexes, Sas-4-N190 or Sas-4-Δ90 remain only in low-density fractions. When mixed with stripped centrosomes, Sas-4 complexes and Sas-4-Δ90 but not Sas-4-N190 are found in the HD fractions. Excess complexes and proteins remain in the unbound fractions. ( c ) Binding assays of Sas-4-Δ90, CNN or a combination of Sas-4-Δ90 and CNN to stripped centrosomes. LD fractions contain unbound proteins, whereas HD fractions contain stripped centrosomes and proteins bound to them. CNN or Asl alone cannot bind stripped centrosomes. In the presence of Sas-4-Δ90 and stripped centrosomes, CNN and Asl are bound to stripped centrosomes. ( d ) Schematic of the Sas-4 protein domains. Tethering: as Sas-4Δ90 binds to stripped centrosomes while Sas-4-N190 does not, the centrosome-binding domain of Sas-4 appears to be between residues 191 and 901. CNN, Asl, β-tubulin binding depends on the presence of the PN2-3 domain. D-PLP and γ-tubulin binding: as Sas-4-N190 binds to D-PLP and γ-tubulin, these proteins' binding domain in Sas-4 appears to be between residues 1 and 190. Green box: conserved segment in PN2-3 domain. CP-190 binding: as Sas-4-N190 and Sas-4Δ150 bind to CP-190, the CP-190 domain of Sas-4 appears to be between residues 151 and 190. ( e ) A model for the role of Sas-4 in PCM formation. Centrosome biogenesis begins with the formation of a nascent procentriole and the assembly of centriole microtubules. S-CAP complexes form in the cytoplasm and are then tethered to a procentriole via Sas-4. The centriole elongates and matures to a functional centrosome. Sas-4 (blue); microtubules (green); PCM (grey); appendages (orange). Full size image In the absence of stripped centrosomes, S-CAP complexes exist solely in the low-density fraction ( Fig. 7b ). Importantly, when we mixed S-CAP complexes with stripped centrosomes, S-CAP complex components are now present in the high-density fraction ( Fig. 7b ). Thus, all factors necessary for binding of a S-CAP complex to stripped centrosomes are present in the cell-free system. In other words, one (or more) of the proteins present in the S-CAP complex is sufficient for directly binding to a stripped centrosome. We then investigated whether Sas-4 is responsible for binding S-CAP complexes to a stripped centrosome. To this end, we purified recombinant Sas-4-N190 (which includes Sas-4's residues 1–190) and Sas-4-Δ90 (which includes residues 90–900), and tested their ability to bind stripped centrosomes ( Supplementary Figs S8b,c and S9a ). In the absence of stripped centrosomes, Sas-4-N190 or Sas-4-Δ90 exists in the low-density fraction ( Fig. 7b ). When we mix Sas-4-N190 and stripped centrosomes, Sas-4-N190 remains in the low-density fraction ( Fig. 7b ), indicating that the first 190 residues of Sas-4 are insufficient for binding stripped centrosomes. However, we find that Sas-4-N190 binds intact centrosomes ( Supplementary Fig. S9b ). Thus, Sas-4's N-terminal domain is sufficient for binding a centrosome component that is absent from stripped centrosomes. Finally, when we mix Sas-4Δ90 and stripped centrosomes, Sas-4Δ90 is found in the high-density (centriolar) fraction, indicating that this Sas-4 variant binds stripped centrosomes ( Fig. 7b ). We then investigated whether Sas-4 tethers CNN and Asl to a stripped centrosome. To this end, we purified recombinant Sas-4Δ90 (which includes the domains that bind CNN, Asl and centrioles), CNN and Asl, and tested their ability to bind stripped centrosomes. In the absence of stripped centrosomes, Sas-4Δ90, CNN or Asl (when mixed or separate) exists in low-density fractions ( Fig. 7c ). Similarly, when we mix CNN, Asl and stripped centrosomes, CNN and Asl remain in the low-density fraction ( Fig. 7c ), indicating that neither protein can bind stripped centrosomes. However, when we mix Sas-4Δ90, CNN, Asl and stripped centrosomes, CNN and Asl are now found in the high-density fraction ( Fig. 7c ). Thus, Sas-4 is able to tether CNN and Asl to a stripped centrosome. These cell-free experiments demonstrate that Sas-4 is responsible for holding S-CAP complex components to the stripped centrosome. Although it is unclear whether Sas-4 binds to the centriole or to the centrosome matrix, these experiments strengthen our hypothesis that S-CAP complex components are tethered in a centrosome via Sas-4. It is known that Sas-4 is necessary for two aspects of centrosome biogenesis: centriole formation and PCM assembly. In centriole formation, without Sas-4, no microtubules are observed and when Sas-4 is overexpressed, microtubules are excessively elongated [26] , [28] , [29] , [30] . Similarly, without Sas-4, PCM does not assemble around a centriole and when Sas-4 is overexpressed, acentriolar PCM-like structures are observed [26] , [27] . The mechanisms by which Sas-4 contributes to the two above-mentioned aspects of centrosome biogenesis had not been demonstrated. The current study shows that Sas-4 performs two major functions during PCM assembly: first, Sas-4 scaffolds cytoplasmic S-CAP complexes by binding to Asl, CNN, D-PLP and CP-190 via its N-terminal domain; second, Sas-4 tethers S-CAP complexes in the centrosome via its C-terminal domain ( Fig. 7d ). Additionally, we discovered that the role of Sas-4 in the centriole formation is independent of its role in PCM assembly. The current findings advance our knowledge of centrosome biogenesis and provide an explanation for the link between it and the human disorder microcephaly. Autosomal recessive primary microcephaly (MCPH) is a disorder where brain size is severely reduced and is caused by mutations in various PCM proteins, for example, Sas-4/CPAP/MCPH6, CNN/MCPH3 and Asl/MCPH4 (refs 46 , 47 ). Another disorder characterized by microcephaly, Seckel syndrome, is caused by mutations in pericentrin (the mammalian D-PLP orthologue) [48] . Recently, patients afflicted with Seckel syndrome were found to bear mutations in sas-4/CPAP and asl/cep152 (refs 49 , 50 ). This new information establishes a common aetiology for primary microcephaly and Seckel syndrome. Perhaps, the MCPH and Seckel syndrome proteins operate together, in a common multi-protein complex and improper assembly or function of that complex underlies the disorders characterized by microcephaly. This explanation is consistent with the findings presented here, which demonstrate that the orthologous MCPH and Seckel syndrome proteins form into S-CAP complexes. The presence of orthologous S-CAP complexes ought to be identified and studied in mammalian brain cells. We have previously shown that Asl and its orthologue Cep152 are critical early in centriole formation [14] . However, Asl is also known to have a role in PCM assembly as the amount of PCM is reduced in Asl's absence [12] , [14] . Recently, a model was proposed that Asl/Cep152 is a scaffold for both Plk4 and Sas-4/CPAP [13] , [20] . According to that model, Asl facilitates centriole formation through its interaction with Plk4 and PCM assembly through its interaction with Sas-4/CPAP. However, the data described in the current work suggest that Sas-4 is responsible for assembling S-CAP complexes that include Asl. Furthermore, certain mutations in Sas-4 prevent the assembly of the S-CAP complexes, suggesting that Sas-4 serves as the scaffold for these complexes. Once a centriole has formed, Sas-4 delivers proteins found at the vicinity of the centriole (including Asl) and tethers them in that location [13] , [14] , [19] . We consider it unlikely that the population of Asl that is recruited to the centrosome by Sas-4 is critical for centriole duplication, as centriole duplication was not eliminated when the levels of Asl in the centrosome were diminished by the Sas-4ΔPN2-3 mutation. An updated model of centrosome biogenesis, which incorporates the findings of this study, is diagrammed in Fig. 7e . Centrosome biogenesis is initiated by Asl and Plk4 (refs 14 , 19 , 20 , 51 ). Later, Sas-6 assembles into a nascent procentriole [26] , [36] , [40] , [43] . In the procentriole, Sas-4 and γ-tubulin ring complexes are involved in microtubule nucleation and elongation [26] , [32] , [52] , [53] . In the cytoplasm, Sas-4 binds to multiple proteins, including CNN, Asl and D-PLP, and serves as the scaffold for the resulting S-CAP complexes. The S-CAP complex is then tethered to a procentriole via Sas-4 molecules present in the complex. These last two steps provide a layer of PCM to the centriole [26] , [28] , [29] , [30] . The centriole then elongates and associates with appendages [54] , [55] . In later phases, more PCM is added to produce functional centrosome [7] , [25] , [48] , [56] , [57] . Plasmids and flies Transgenic flies and Sas-4 constructs were previously described [14] , [21] . P[lacW]l(3)s2214 (Sas-4s2214) was obtained from the Bloomington Stock Center. GST-CNN was constructed by insertion of a Kpn I– Sal I fragment of cnn-RA cDNA into the Kpn I– Sal I site of pGEX2 (Stratagene). The resulting plasmid expresses amino acids 17–1,148 of CNN-PA with GST at its amino terminus. GST-CNN-N and GST-CNN-C were PCR amplified and cloned into pGEX2 to produce plasmids that express CNN's amino acids 17–558 and 517–1,048, respectively. Sas-4 cDNA (GM21734) was obtained from the Berkeley Drosophila Genome Project. For Sas-4-C90, amino acids 90–900 was amplified from Sas-4 cDNA and cloned into pET24B that express Sas-4-C90 as HIS-tagged fusion protein. Sas-4-N190 was a generous gift from the Tang lab. For Sas-4-N190ΔPN2-3, the PN2-3 domain was deleted from Sas-4-N190 and cloned into pGEX2. For Sas-4ΔPN2-3, the PN2-3 domain was deleted from Sas-4 cDNA by using Quick change exchange kit (Stratagene). All Sas-4 constructs for in vivo expression were subcloned into pUAS vectors in a manner that the cloned proteins were expressed using a Sas-4 promoter rather than overexpressed using the GAL4 system. Drosophila embryonic and S2 cell extracts A 0–8-h Drosophila embryo extracts were prepared as described [4] . Briefly, embryos were homogenized in extract buffer containing 80 mM K-PIPES, pH 6.8, 1 mM MgCl 2 , 1 mM Na 3 EGTA, 14% sucrose, 100 mM KCl, 1 mM PMSF, protease inhibitor cocktail and EDTA-free Roche complete tablets (Roche). The crude extract was centrifuged for 20 min at 1,500 g at 4° C to obtain a low-speed lysate, which contained centrosomes and cytoplasmic complexes. A HSL was prepared similarly but was instead centrifuged for 30 min at 200,000 g . Similar procedures were used for Drosophila S2 cells. Stable Drosophila S2 cell lines that express variants of Sas-4 were established by co-transfecting plasmids containing a Sas-4 construct with a hygromycin-resistant plasmid (Invitrogen). Purification of native Sas-4 complexes Protein G beads were coated with an anti-Sas-4 or anti-GFP (Roche) antibody overnight at 4° C. The antibody-coated beads and embryonic/S2 extracts were mixed and incubated at 4° C for 4 h, twice washed with extract buffer containing 0.1% Triton X-100, and then twice washed with extract buffer. The beads were eluted by boiling in Laemmli sample buffer. Recombinant Sas-4-N190 (35 μM) was used to purify native Sas-4 complexes. For TAP purification, HSL was incubated with IgG-coated beads, the bound product was TEV cleaved, and the Sas-4 complexes were bound to calmodulin beads. The complexes were eluted in buffer containing 10 mM EGTA. For GST pull downs, the bait was recombinant Sas-4-N-GST or Sas-4-N190ΔPN2-3 bound to GST agarose and the source of Sas-4-N190 was embryonic HSL; 20 mM glutathione was used for the elution. When required, an anti-GFP antibody (Roche) was used for the co-immunoprecipitation experiments. Sucrose gradient velocity sedimentation Sucrose was dissolved in extract buffer including either 100 or 500 mM KCl. Continuous gradients of 15–60% were generated with a Gradient Master (Biocomp). Centrifugation at 243,000 g for 13 h at 4 °C was performed using an SW-40 rotor (Beckman Coulter). Liquid chromatography MS/MS Protein samples were in-solution trypsinized. Tryptic peptides were analysed by liquid chromatography MS/MS. Peptides were separated across a 45-min gradient ranging from 10 to 35% (v/v) acetonitrile in 0.1% (v/v) formic acid in a microcapillary (125 μm×18 cm) column packed with C18 reverse-phase material: Magic C18AQ, 5 μm particles, 200 Å pore size (Michrom Bioresources). The peptides were analysed using an LTQ XL linear ion trap mass spectrometer (ThermoFisher). For each cycle, one full MS scan was followed by ten MS/MS spectra from the ten most abundant ions. MS/MS spectra were searched using the Sequest algorithm against a Drosophila protein database. All peptide matches were filtered based on tryptic state, Xcorr and dCorr. Western blotting Samples were resolved in 8% acrylamide gels or 3–12% gradient gels for D-PLP. Proteins were transferred to nitrocellulose membranes and incubated with primary antibodies overnight at 4 °C followed by secondary antibodies at room temperature for 1 h. Super Signal West Pico or Femto Chemilluminescent substrate (Pierce) detected peroxidase activity. Molecular masses were determined by comparison with ProSieve molecular standards (Lonza). The apparent molecular weights of proteins detected by specific antibodies were Sas-6: 54 kDa, Asl: 115 kDa, CNN: 150 kDa, Sas-4: 100 kDa, CP-190: 190 kDa and tubulin: 50 kDa. Antibodies A cDNA fragment containing amino acids 2–150 of Drosophila Sas-4 was cloned into a pET vector (Invitrogen) and expressed in Escherichia coli. Inclusion bodies were prepared and resolved using SDS–polyacrylamide gel electrophoresis. Protein was extracted from the gel and injected into mice. Hybridomas were prepared and the monoclonal antibody was collected using standard protocols. For western blots, the monoclonal mouse anti-Sas-4 (1:500), rabbit anti-CNN (1:5,000, courtesy of C. Kaufman), mouse anti-γ-tubulin (1:5,000, Sigma-Aldrich), mouse anti-GFP (1:5,000, Roche), mouse or rabbit anti-β-tubulin (1:5,000, Sigma), rabbit anti-Sas-6 (1:5,000, Gopalakrishnan et al . [36] ), rabbit anti-Asl (1:5,000, Blachon et al . [14] ), rabbit anti-D-PLP (1:1,000, courtesy of J. Raff), rabbit anti-CP-190 (1:5,000, courtesy of V. Corces) and rabbit anti-Plk4 (1:5,000, courtesy of M. Bettencourt). Peroxidase-conjugated secondary antibodies were used at 1:5,000 (Vector Labs). For immunofluorescence, rat anti-α-tubulin (1:200, Chemicon), mouse anti-γ-tubulin (1:200), the above-described monoclonal mouse anti-Sas-4 (1:100), rabbit anti-CNN (1:200), rabbit anti-D-PLP (1:200), rabbit anti-Asl (1:200), and rabbit anti-CP-190 (1:200) were used. Secondary antibodies Cy5 goat anti-mouse and rhodamine donkey anti-rat were used at 1:200 (ImmunoResearch). 4,6-diamidino-2-phenylindole (DAPI) (1 μg ml −1 , Sigma) stained DNA. Immuno-microscopy Drosophila S2 cells were grown on concanavalin A-coated cover slips for 1 h at 25 °C and then fixed with formaldehyde (3.7% in PBS) for 5 min. Cells were permeabilized with 0.1% Triton X-100 in PBS for 10 min and blocked with 1% BSA, 0.1% Triton X-100 in PBS for 45 min. Antibody labelling was performed for 1 h at room temperature followed by three washes in PBS. A similar protocol was used for testes labelling. Confocal images were collected using a Leica TCS SP5 scanning confocal microscope; 3D-SIM images were collected using the DeltaVision|OMX microscope [33] . Images were processed using Adobe Photoshop. Immuno-electron microscopy was performed as described [14] , [36] . Recombinant proteins Sas-4-N190, Sas-4-N190ΔPN2-3, Sas-4Δ-90, CNN and Asl proteins were expressed in Escherichia coli strain BL21(DE3)pLysE via isopropylthiogalactoside induction. The soluble fraction of Sas-4-N190 or Sas-4-N190ΔPN2-3 was purified using GST-agarose affinity beads. For CNN and Sas-4-Δ90, cells were sonicated and inclusion bodies were pelleted by centrifugation for 30 min at 18,500 g . Inclusion bodies were twice homogenized in 1% Triton X-100, 1 M urea, 100 mM Tris buffer pH 7, 5 mM EDTA and centrifuged at 18,500 g . The homogenized inclusion bodies were washed in 100 mM Tris pH 7, 5 mM EDTA, suspended in 20 mM Tris pH 7.5, 100 mM NaCl, 8 M urea, 10 mM 2-mercaptoethanol, and dialysed against progressively decreasing urea, in 1 M steps, with, at least, 1 h between steps. The refolded proteins were dialysed against 20 mM Tris pH 7.5, 100 mM NaCl, 30% glycerol. Sas-4-Δ90 was purified similarly yet with the step involving 8 M urea omitted. The affinity-purified protein was then dialysed against 20 mM Tris pH 7.5. Recombinant proteins were then subjected to size exclusion using Superose 12 column, and the purified peak fractions were collected. Centrosome binding assay To assay the ability of a Sas-4 complex or recombinant Sas-4-N190, Sas-4-Δ90, CNN or Asl to bind to centrosomes or to stripped centrioles, discontinuous sucrose gradient sedimentation was used. SW-55 tubes (Beckman) were cushioned with 300 μl 70% sucrose followed by 40% sucrose, both in extract buffer having 100 mM KCl (described above). Sas-4 complexes or recombinant Sas-4 proteins were mixed with centrosomes or stripped centrosomes to a volume of 4 ml in the presence of 1 mM GTP and mixed for 4 h at 4 °C. This mixture was layered on the 40% sucrose cushion and was spun in an SW-55 rotor at 300,000 g for 1 h. Fractions were collected from the bottom of the gradient by puncturing the tube with an 18.5-gauge needle. The first three fractions (250 μl each), the next five fractions (500 μl) and a final fraction (the remaining volume) were collected. The first two fractions, that is, the high-density fractions, contained centrosomes with bound proteins; the final fraction, that is,, the low-density fraction, contained only unbound proteins. How to cite this article: Gopalakrishnan, J. et al . Sas-4 provides a scaffold for cytoplasmic complexes and tethers them in a centrosome. Nat. Commun. 2:359 doi: 10.1038/ncomms1367 (2011).